Photolatently modulable hydrogels using unilamellar titania nanosheets as photocatalytic crosslinkers Hydrogels, postmodulable in controlled time and space domains, attract particular attention due to their potential in bio-related applications. Towards this goal, photolatently reactive hydrogels are very promising. Here we develop photolatently modulable hydrogels, composed of a polymer network accommodating photocatalytic titania nanosheets at every crosslinking point. As titania nanosheets can utilize gelling water as their source of radicals, its long-lasting photocatalysis makes the hydrogels readily modulable. Benefiting from the hydrogelation mechanism, the gel network is finely compartmentalized, leading to sharp thermoresponses. As demonstrated by photo-micropatterning, non-diffusible titania nanosheets at the crosslinking points enable pointwise modulations with an excellent spatial resolution. The photolatent nature also makes it possible to conjugate them with other hydrogels and polymers. With increasing demand for human- and environment-friendly renewable materials, particular attention has been focused on hydrogels, a class of soft matter mainly composed of water [1] , [2] , [3] , [4] , [5] , [6] . Meanwhile, hydrogel materials, whose structures and functions are postmodulable multiple times, just like living tissues, have long been awaited [7] , [8] , [9] , [10] . Indeed, various applications are expected for hydrogels that are modulable noninvasively in desired time and space domains [11] , [12] , [13] , [14] , [15] , [16] . Towards this goal, photolatently reactive hydrogels that can be activated by light are most promising. Ideally, such hydrogels are dormant under ambient conditions but quickly activated by exposure to light, to enable localized postmodulations. Recently, two-dimensional nanosheets [17] , [18] , [19] , [20] have caught special attention as components of hydrogels. In 2002, Haraguchi and Takehisa [17] reported that radical polymerization of vinyl monomers in an aqueous colloidal dispersion of disk-shaped clay nanosheets (Laponite XLG) gives rise to mechanically tough nanocomposite hydrogels. More recently, we reported that, upon mixing with Laponite, poly(ethylene glycol) derivatives featuring adhesive dendronized termini, allow for the formation of strong noncovalent hydrogels [18] . In these cases, clay nanosheets physically crosslink polymer chains, in situ generated or externally added, and ensure the formation of a strong three-dimensional polymer network for holding water molecules inside. We envisioned that the use of unilamellar titania nanosheets, instead of Laponite, may provide modulable hydrogels with photolatently reactive crosslinking points ( Fig. 1 ). 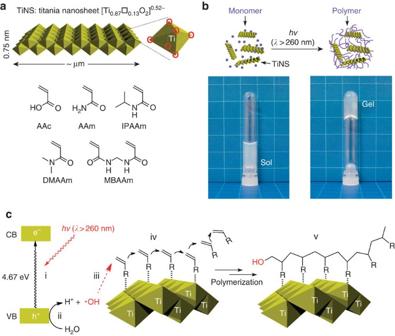Figure 1: Light-mediated hydrogelation. (a) Schematic structure of TiNS and list of vinyl monomers used for photoinduced hydrogelation. (b) Schematic illustration of TiNSs (0.4 wt%)-mediated photoinduced hydrogelation (λ>260 nm, at 25 °C for 20 min) and pictures before and after the hydrogelation using IPAAm(10.0 wt%) as monomer. (c) Expected elementary steps involved in photoinduced hydrogelation: (i,ii) photocatalytic generation of a hydroxyl radical by TiNSs from water; (iii,iv)in situpolymerization of vinyl monomers by the photogenerated hydroxyl radical; (v) physical crosslinking of polymer chains by TiNSs via noncovalent interactions. Figure 1: Light-mediated hydrogelation. ( a ) Schematic structure of TiNS and list of vinyl monomers used for photoinduced hydrogelation. ( b ) Schematic illustration of TiNSs (0.4 wt%)-mediated photoinduced hydrogelation ( λ >260 nm, at 25 °C for 20 min) and pictures before and after the hydrogelation using IPAAm(10.0 wt%) as monomer. ( c ) Expected elementary steps involved in photoinduced hydrogelation: (i,ii) photocatalytic generation of a hydroxyl radical by TiNSs from water; (iii,iv) in situ polymerization of vinyl monomers by the photogenerated hydroxyl radical; (v) physical crosslinking of polymer chains by TiNSs via noncovalent interactions. Full size image Titania is a renowned photocatalyst that has been studied extensively [21] , [22] , [23] . Upon exposure to ultraviolet light in water, titania is photoexcited to generate an electron/hole pair, the latter of which oxidizes water, producing a hydroxyl radical efficiently [24] , [25] , [26] . In 1996, the group of Sasaki et al . [27] , a coauthor of the present work, reported the first successful exfoliation of layered titania into unilamellar titanate nanosheets (TiNSs) in aqueous media. As illustrated in Fig. 1a , TiNS is ultrathin (0.75 nm thick) and negatively charged, where all titanium and oxygen atoms are exposed on the surface and arranged two-dimensionally to furnish a single-crystal-like order [28] , [29] , [30] ( Supplementary Table S1 ). Here we report that the use of TiNSs as a photocatalytic crosslinker, in conjunction with appropriate water-soluble vinyl monomers, allows for one-step preparation of photolatently modulable hydrogels. The gels can be activated whenever exposed to light, and generate hydroxyl radicals for postmodulation ( Fig. 1c ). As the photocatalytic activity of TiNS is long lasting, our hydrogels work multiple times using light and water in the gel matrix. Equally important, photocatalytic TiNSs are immobilized at the crosslinking points, thereby enabling pointwise photo-modulations with an excellent spatial resolution. As exemplified in the present work, the photolatently modulable hydrogels, readily preparable using photocatalytic TiNSs as a crosslinker, are promising for various applications. Preparation and thermoresponses of hydrogels The photolatently modulable hydrogels were prepared as follows. Typically, TiNSs (0.4 wt%) were dispersed in an aqueous solution of a water-soluble vinyl monomer such as N -isopropylacrylamide (IPAAm, 10 wt%) ( Fig. 1a ), and the resultant translucent dispersion was exposed to light ( λ >260 nm) from a 500-W mercury arc lamp for 20 min at room temperature (~25 °C), wherein radical polymerization of IPAAm took place, affording a translucent hydrogel ( Fig. 1b ). Its rheological properties ( Supplementary Fig. S1 and Supplementary Methods ) were typical of ordinary hydrogels. We found that this hydrogel sharply and reversibly changes, without any hysteresis, its optical transmittance in a very narrow temperature range of 32–33 °C ( Fig. 2c ). When the hydrogel, processed into a 50-μm-thick film, was heated abruptly from 32 to34 °C, its optical transmittance fell in just 3 s from 86 to 0% ( Fig. 2d , blue curve). Cooling back to 32 °C allowed the hydrogel film to quickly recover its original transparency ( Fig. 2d , blue curve and Supplementary Methods ). In aqueous media, poly(IPAAm) is hydrated by a dipole–dipole interaction. However, upon heating above 32 °C, the polymer chains are dehydrated and aggregate together, eventually forming a precipitate [31] , [32] , [33] , [34] . This is known as the lower critical solution temperature (LCST) phenomenon, which certainly accounts for the temperature-dependent optical transmittance change in Fig. 2c . As demonstrated in Fig. 2b , the hydrogel prepared with the TiNS crosslinker (IPAAm/TiNSs=10.0/0.4 wt%) remained sharply thermoresponsive even when integrated into a patterned poly(dimethylsiloxane) (PDMS) matrix. In accordance with the literature [35] , we employed an organic crosslinker ( Fig. 1a ; N , N ′-methylenebis(acrylamide) (MBAAm), 0.1 wt%), instead of TiNSs, for the preparation of a reference hydrogel film ( Supplementary Methods ). As exemplified by this reference sample, organically crosslinked poly(IPAAm)-based hydrogels, without any particular design [36] , [37] , generally show a very poor and sluggish thermoresponse in optical transmittance ( Fig. 2d , red curve). 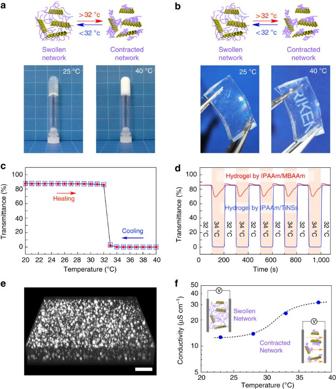Figure 2: Thermoresponsive behaviours of hydrogels. (a,b) Pictures of a hydrogel prepared with IPAAm/TiNSs (10.0/0.4 wt%) at 25 and 40 °C in a test tube (a) and in a patterned PDMS matrix (b). (c) Transmittances (300 nm) of a 50-μm-thick film of the hydrogel at different temperatures in the range 20–40 °C, where the data with red filled circles and blue open squares are for the heating and cooling processes, respectively. (d) Time-dependent transmittance (300 nm) changes of a 50-μm-thick film sample of the hydrogel (blue curve) and those of a reference hydrogel (red curve) prepared with MBAAm as the crosslinker (IPAAm/MBAAm=10.0/0.1 wt%) in response to repeated temperature jump/drop cycles in the range 32–34 °C. (e) A three-dimensional microstructure of the hydrogel constructed with its sliced two-dimensional images, obtained at 34 °C by confocal fluorescence laser scanning microscopy, where the sample was doped with a fluorescent probe (8-anilino-1-naphthalenesulphonic acid ammonium salt). Scale bar, 10μm. (f) Ion conductivities of the hydrogel at different temperatures in the range 23–38 °C at an applied cell voltage of 100 mV, where the sample was doped with LiClO4(500 mM). Figure 2: Thermoresponsive behaviours of hydrogels. ( a , b ) Pictures of a hydrogel prepared with IPAAm/TiNSs (10.0/0.4 wt%) at 25 and 40 °C in a test tube ( a ) and in a patterned PDMS matrix ( b ). ( c ) Transmittances (300 nm) of a 50- μ m-thick film of the hydrogel at different temperatures in the range 20–40 °C, where the data with red filled circles and blue open squares are for the heating and cooling processes, respectively. ( d ) Time-dependent transmittance (300 nm) changes of a 50-μm-thick film sample of the hydrogel (blue curve) and those of a reference hydrogel (red curve) prepared with MBAAm as the crosslinker (IPAAm/MBAAm=10.0/0.1 wt%) in response to repeated temperature jump/drop cycles in the range 32–34 °C. ( e ) A three-dimensional microstructure of the hydrogel constructed with its sliced two-dimensional images, obtained at 34 °C by confocal fluorescence laser scanning microscopy, where the sample was doped with a fluorescent probe (8-anilino-1-naphthalenesulphonic acid ammonium salt). Scale bar, 10 μ m. ( f ) Ion conductivities of the hydrogel at different temperatures in the range 23–38 °C at an applied cell voltage of 100 mV, where the sample was doped with LiClO 4 (500 mM). Full size image The ultra-sharp thermoresponse, thus revealed for our TiNS-mediated hydrogel, is most likely given by its finely compartmentalized microstructure. For visualizing its microstructure, a fluorescent probe (8-anilino-1-naphthalenesulphonic acid ammonium salt) that luminesces only in hydrophobic environments [38] was doped into a hydrogel prepared with IPAAm/TiNSs (10.0/0.4 wt%). At a temperature above LCST, the hydrogel with an opaque appearance, in confocal laser scanning microscopy ( Supplementary Methods ), indeed displayed a large number of submicron-sized tiny luminescent domains ( Fig. 2e ). This fine compartmentalization, which is advantageous for quick thermal shrinkage/swelling of polymer domains, certainly benefits from the mechanism of hydrogelation with photocatalytic TiNSs. In the initial stage of hydrogelation, the IPAAm monomer polymerizes mostly around TiNSs with hydroxyl radicals locally photogenerated. As a result, produced polymer chains are kinetically trapped by proximal TiNSs and compartmentalized before they grow up to assemble a large polymer domain ( Fig. 1c ). With this structure-driven sharp LCST behaviour, our hydrogel can act as a thermoresponsive ion gate ( Fig. 2f and Supplementary Methods ). For this purpose, a hydrogel prepared with IPAAm/TiNSs (10.0/0.4 wt%) was doped with LiClO 4 upon immersion for 2 days in an aqueous solution of LiClO 4 (500 mM). This electrolyte-doped hydrogel showed a general trend with higher ion conductivity at higher temperature ( Fig. 2f and Supplementary Fig. S2 ). However, at a closer look, its ion conductivity increased markedly at around the LCST. For example, the change in conductivity from 28 to 33 °C is 4.5 times greater than that from 23 to 28 °C and 2.9 times greater than that from 33 to 38 °C. Again, this thermoresponsive ion-gating feature is provided by the sharp LCST behaviour that benefits from the finely compartmentalized polymer domains in the hydrogel matrix. The TiNS surface bears Ti-O − groups ( Fig. 1a ). For the hydrogelation with photocatalytic TiNSs, vinyl monomers with a certain affinity towards negatively charged TiNS are effective ( Fig. 1a ) [39] . In addition to the IPAAm described above, acrylamide (AAm) and acrylic acid (AAc), both having a proton-donating ability, led to successful hydrogelation. In contrast, the use of N , N -dimethylacrylamide (DMAAm), with no capability of proton donation, resulted in a considerably weak hydrogel. In consistency with this hypothesis, 1 H NMR signals (in D 2 O at 25 °C) of IPAAm (8.0 wt%) significantly broadened when mixed with a minute amount of TiNSs (0.4 wt%), whereas those of DMAAm (8.0 wt%) hardly changed ( Supplementary Fig. S3 and Supplementary Methods ). Also noteworthy, even when polymers are affinitive to TiNSs such as poly(IPAAm), no hydrogel but a heterogeneous viscous fluid is formed upon mixing TiNSs with those polymers that are separately prepared. This observation indicates that the hydrogelation occurs kinetically, most likely because TiNSs, responsible for the in situ polymer formation, also act as a physical crosslinker for the produced polymer chains ( Fig. 1c ). For hydrogelation, we also found that the use of photocatalytic TiNSs in conjunction with Laponite works for a broader range of monomers including DMAAm having a poor affinity towards TiNSs. Laponite does not deteriorate the photocatalysis of TiNSs, but possibly helps the crosslinked polymer network to be more reinforced and widely developed [17] , [18] . Micropatterning of hydrogels In our hydrogel, TiNSs are presumably fixed at the crosslinking points in a three-dimensional polymer network and therefore hardly diffuse inside the gel matrix. Hence, photocatalytic events by TiNSs in the gel matrix may be performed pointwise with an excellent spatial resolution. With this possibility in mind, we attempted micropatterning of our hydrogel by using its photolatent reactivity [11] , [12] , [40] . Thus, a hydrogel prepared with DMMAm/TiNSs (8.0/3.0 wt%), in conjunction with Laponite (3.0 wt%), was immersed in an aqueous solution of IPAAm (8.0 wt%) and after shortly washing its surface, the resultant hydrogel was exposed to light ( λ >260 nm) for 20 min through a micropatterned photomask (500 × 500 μm 2 open squares). The hydrogel consisting of a DMMAm polymer network does not display any LCST behaviour. Therefore, if poly(IPAAm), active for LCST, is formed pointwise, one may observe polymer domains that selectively scatter light upon heating. As shown in Fig. 3b , the heated hydrogel, obtained after the light exposure, indeed displayed a micropattern with analogous configuration and spatial resolution to those of the photomask. Although the lifetime of a hydroxyl radical in water is quite short (10 −5 s) (ref. 41 ), a growing carbon radical in water has been reported to live longer in a range of 10 −1 –10 0 s and is, in principle, diffusible in a gel matrix. Nevertheless, as described already, both the monomer and polymer interact with TiNSs strongly. When hydroxyl radicals are generated by photoexcited TiNSs, the polymerization most likely proceeds in close proximity to TiNSs ( Supplementary Fig. S3 ), where the resultant polymer chains are kinetically trapped by TiNSs and not allowed to diffuse freely. As a consequence of this, the growing polymer radicals are locally concentrated, so that the probability of their recombination is enhanced. We suppose that this is why the hydrogel can be micropatterned with an excellent spatial resolution. For further expansion of this achievement, we attempted photo-micropatterning using the reduction of Ag + into Ag nanoclusters [42] , [43] . Again, immobilized TiNSs, upon light exposure, allowed for successful replication of the masked pattern in the hydrogel matrix with black dots ( Fig. 3c ). By using a photomask with a much larger pattern (2-mm-wide open circles), we confirmed that the black dots show a surface-plasmonic absorption centreed at 500 nm due to Ag nanoclusters ( Supplementary Fig. S4 ). As shown in Fig. 3d , this absorption became monotonically stronger as the exposure time was longer, but the outline of the micropattern did not become vague ( Fig. 3d , insets). 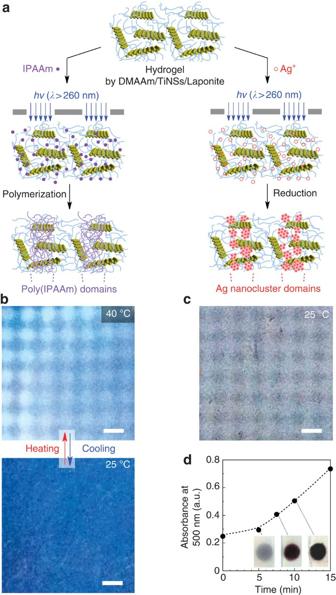Figure 3: Micropatterning of photolatently modulable hydrogels. (a) Schematic illustration of micropatterning with poly(IPAAm) and Ag nanocluster in a hydrogel matrix, prepared with DMAAm/TiNSs/Laponite (8.0/3.0/3.0 wt%), upon light exposure (λ>260 nm) through a patterned photomask (500 × 500 μm2open squares). (b) Pictures of a micropatterned hydrogel with poly(IPAAm) at 40 and 25 °C. Scale bar, 500 μm. (c) A picture of a micropatterned hydrogel with Ag nanocluster at 25 °C. Scale bar, 500 μm. (d) Change in surface plasmonic absorbance (500 nm) with light exposure time of Ag nanocluster micropatterned in the hydrogel. Figure 3: Micropatterning of photolatently modulable hydrogels. ( a ) Schematic illustration of micropatterning with poly(IPAAm) and Ag nanocluster in a hydrogel matrix, prepared with DMAAm/TiNSs/Laponite (8.0/3.0/3.0 wt%), upon light exposure ( λ >260 nm) through a patterned photomask (500 × 500 μm 2 open squares). ( b ) Pictures of a micropatterned hydrogel with poly(IPAAm) at 40 and 25 °C. Scale bar, 500 μm. ( c ) A picture of a micropatterned hydrogel with Ag nanocluster at 25 °C. Scale bar, 500 μm. ( d ) Change in surface plasmonic absorbance (500 nm) with light exposure time of Ag nanocluster micropatterned in the hydrogel. Full size image Homo- and heterotropic conjugations of hydrogels The photocatalytic activity of crosslinking TiNSs allows our hydrogels to be conjugated with other objects homo- and heterotropically, so long as the gels contain a monomer in addition to water, the source of hydroxyl radicals. As shown in Fig. 4a , we processed a rod-shaped object from a hydrogel, prepared with DMMAm/TiNSs (8.0/3.0 wt%) in conjunction with Laponite (3.0 wt%), and chopped it into two pieces. Then, one piece at its chopped surface was treated with a small amount of DMAAm (~20 μl cm −2 ), and then the two pieces were put together in such a way that their chopped surfaces came into contact with each other. After light exposure ( λ >260 nm) for 20 min, the two pieces merged perfectly, affording a single rod without any visible history of the breakage ( Fig. 4a ). Note that, without light exposure, they did not merge under identical conditions. In a tensile test, the photo-conjugated rod-shaped object could be stretched without breakage up to an applied strain of 500% ( Fig. 4b and Supplementary Methods ). Even more challenging is to realize heterotropic conjunction. For this purpose, we prepared a rod-shaped object from PDMS ( Fig. 4d ) and likewise tested the possibility of heterotropic conjunction with our photolatently modulable hydrogel ( Fig. 4d ). As shown in Fig. 4d , the two rods merged completely after light exposure ( λ >260 nm) for 20 min, where the resultant single-rod object did not break up until the applied strain reached 550% ( Fig. 4e ). Heterotropic hydrogel/hydrogel and hydrogel/polymer conjunctions possibly expand the potential of our modulable hydrogels. For example, lateral photochemical conjunction of two hydrogel strips with different thermoresponsive properties provides a soft actuator that operates by a temperature change ( Supplementary Fig. S5 and Supplementary Methods ) [44] , [45] , [46] . 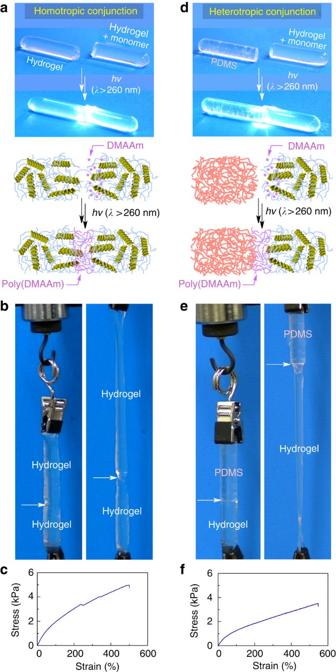Figure 4: Homo- and heterotropic conjugations of photolatently modulable hydrogels. (a–c) Homotropic conjugation of chopped hydrogel rods prepared with DMAAm/TiNSs/Laponite (8.0/3.0/3.0 wt%). A picture of the homotropic conjugation process with light (λ>260 nm) (a), pictures of a conjugated rod and its deformation in tensile testing (b), and strain–stress curve (c). (d–f) Heterotropic conjugation of a hydrogel rod with a PDMS rod. A picture of the heterotropic conjugation process with light (λ>260 nm) (d), pictures of a conjugated rod and its deformation in tensile testing (e), and strain–stress curve (f). Figure 4: Homo- and heterotropic conjugations of photolatently modulable hydrogels. ( a – c ) Homotropic conjugation of chopped hydrogel rods prepared with DMAAm/TiNSs/Laponite (8.0/3.0/3.0 wt%). A picture of the homotropic conjugation process with light (λ>260 nm) ( a ), pictures of a conjugated rod and its deformation in tensile testing ( b ), and strain–stress curve ( c ). ( d – f ) Heterotropic conjugation of a hydrogel rod with a PDMS rod. A picture of the heterotropic conjugation process with light (λ>260 nm) ( d ), pictures of a conjugated rod and its deformation in tensile testing ( e ), and strain–stress curve ( f ). Full size image By using titania, one of the most reputed and thoroughly studied inorganic semiconductors, we developed ‘photolatently modulable’ hydrogels that are readily preparable and also postmodulable by light whenever needed. The titania TiNS we employed here adopts a sheet shape ( Fig. 1a ), which has a dual role in hydrogelation: (1) generating hydroxyl radicals from water for inducing radical polymerization and (2) kinetically crosslinking the produced polymer chains to form a three-dimensional polymer network for holding water molecules inside. Consequently, TiNSs are immobilized at the crosslinking points in a polymer network and locally convert gelling water into hydroxyl radicals whenever exposed to light. The diffusionless photocatalysis, realized by using crosslinking TiNSs, allows for pointwise hydrogel modulations when coupled with top-down fabrication techniques. Also noteworthy, the photocatalytic activity of titania is long lasting, in contrast with those of organic pigments, and hardly contaminates hydrogels even upon repeated photo-modulation events. Titania is nontoxic and biocompatible, unlike most other inorganic semiconductors, and has already been used as an essential component in biomedical devices. Hence, the photolatently modulable hydrogels have the potential for many applications. Future perspectives may include design of multilayered hydrogel spheres for controlled drug release, creation of semi-synthetic enzymes by multistep pointwise co-immobilizations of natural enzymes with synthetic catalysts, and three-dimensional tissue engineering by cultivation of multiple cells in different time and space domains. These challenges would also encourage the development of conceptually new photocatalytic inorganic sheets. Hydrogelation with IPAAm/TiNSs An aqueous dispersion of TiNSs (0.4 wt%) containing IPAAm (10.0 wt%) was exposed at 25 °C to a 500-W high-pressure mercury arc light ( Supplementary Methods ) through a filter to cut off short-wavelength ( λ <260 nm) light, whereupon radical polymerization of IPAAm took place and reached complete consumption of IPAAm in 20 min, affording a hydrogel. According to a procedure analogous to that described above, hydrogelation with other vinyl monomers (AAm, AAc and DMAAm) using TiNSs was conducted. Hydrogelation with IPAAm/TiNS/Laponite To an aqueous dispersion of TiNSs (3.0 wt%) at 25 °C was successively added IPAAm (8.0 wt%) and Laponite XLG (3.0 wt%). The mixture was stirred at 25 °C until Laponite XLG was well dispersed and then exposed at 25 °C to a 500-W high-pressure mercury arc light through a filter to cut off short-wavelength ( λ <260 nm) light, whereupon radical polymerization of IPAAm took place and reached complete consumption of IPAAm in 20 min, affording a hydrogel. According to a procedure analogous to that described above, hydrogelation with other vinyl monomers (AAm, AAc and DMAAm) using TiNSs/Laponite was conducted. Micropatterning of a hydrogel with poly(IPAAm) A hydrogel prepared with DMAAm/TiNSs/Laponite (8.0/3.0/3.0 wt%) was immersed in an aqueous solution of IPAAm (8.0 wt%) for 2 days, and its surface was shortly washed. Through a micropatterned photomask (500 × 500 μm 2 open squares), the resultant hydrogel was exposed at 25 °C for 20 min to a 500-W high-pressure mercury arc light after passing through a filter to cut off short-wavelength ( λ <260 nm) light. Micropatterning of a hydrogel with Ag nanocluster A hydrogel prepared with DMAAm/TiNSs/Laponite (8.0/3.0/3.0 wt%) was immersed in an aqueous solution of AgNO 3 (50 mM) for 2 days, and its surface was shortly washed. Through a micropatterned photomask (500 × 500 μm 2 open squares), the resultant hydrogel was exposed at 25 °C for 20 min to a 500-W high-pressure mercury arc light after passing through a filter to cut off short-wavelength ( λ <260 nm) light. Homotropic conjugation of hydrogels A rod-shaped hydrogel prepared with DMMAm/TiNSs/Laponite (8.0/3.0/3.0 wt%) was cut into two pieces. The cut surface of one piece was treated with a small amount of DMAAm (~20 μl cm −2 ) and then allowed to come into contact with the cut surface of the other piece. The joint region was then exposed at 25 °C for 20 min to a 500-W high-pressure mercury arc light through a filter to cut short-wavelength ( λ <260 nm) light. Heterotropic conjugation of a hydrogel with PDMS One end of a rod-shaped hydrogel prepared from DMAAm/TiNSs/Laponite (8.0/3.0/3.0 wt%) was treated with a small amount of DMAAm (~20 μl cm −2 ), while a PDMS rod was exposed to oxygen plasma at 25 °C for 15 min. Two modified ends were then allowed to come into contact with each other, and the junction region was exposed at 25 °C for 20 min to a 500-W high-pressure mercury arc light through a filter to cut off short-wavelength ( λ <260 nm) light. How to cite this article: Liu, M. et al . Photolatently modulable hydrogels using unilamellar titania nanosheets as photocatalytic crosslinkers. Nat. Commun. 4:2029 doi: 10.1038/ncomms3029 (2013).